Identification of myopia-associated WNT7B polymorphisms provides insights into the mechanism underlying the development of myopia Myopia can cause severe visual impairment. Here, we report a two-stage genome-wide association study for three myopia-related traits in 9,804 Japanese individuals, which was extended with trans-ethnic replication in 2,674 Chinese and 2,690 Caucasian individuals. We identify WNT7B as a novel susceptibility gene for axial length (rs10453441, P meta =3.9 × 10 −13 ) and corneal curvature ( P meta =2.9 × 10 −40 ) and confirm the previously reported association between GJD2 and myopia. WNT7B significantly associates with extreme myopia in a case–control study with 1,478 Asian patients and 4,689 controls (odds ratio (OR) meta =1.13, P meta =0.011). We also find in a mouse model of myopia downregulation of WNT7B expression in the cornea and upregulation in the retina, suggesting its possible role in the development of myopia. High myopia increases the risk of other pathological ocular complications [1] , owing to which myopia is emerging as a major public health concern in many parts of the world. The prevalence of high myopia and associated visual complications is increasing in many Asian and Caucasian populations, and this trend is particularly notable in urbanized areas [2] , [3] , [4] . The World Health Organization recognizes myopia as a major cause of visual impairment [5] . Emmetropia, the absence of refractive error, is determined by the precise coordination of ocular parameters, such as axial length, corneal curvature, lens thickness and anterior chamber depth. Disruption of this coordination causes refractive errors, such as myopia and hyperopia [6] , [7] . Of these components, axial length plays a major role in refraction; therefore, in clinical settings, the degree of myopia is predominantly determined by axial length [8] , [9] , [10] . A recent large-scale, genome-wide meta-analysis by the Consortium for Refractive Error and Myopia (CREAM) reported that 23 of 29 loci associated with refraction were also associated with axial length [11] , [12] . However, genes associated with axial length are not necessarily associated with refractive error [12] . This can be explained on the basis of the compensatory effects of other ocular biometric components, such as corneal curvature that influence the effect of an increased axial length through a flatter cornea [6] . Indeed, in genome-wide association studies (GWASs), some genes found to be associated with corneal curvature were also recently reported to be associated with axial length, but not with refractive error [7] , [13] . On the other hand, the retina is thought to play a crucial role in the development of myopia [14] . For example, it is well known that central hyperopic defocus can cause myopia in chicks [15] and mice models [16] . In addition, experiments conducted by Smith et al. [17] , [18] , [19] have shown that peripheral hyperopic defocus can cause myopic shift in monkeys. This is a herald of ‘peripheral defocus theory’ that implicates defocus at the peripheral retina as the trigger for myopia. These reports suggest that the retina can perceive the defocus and evoke signals to accelerate the progression of myopia. This hypothesis is supported by animal experiments that show amacrine cells and their transcription factor, ZENK, have important roles in the perception of retinal defocus [20] , [21] . Nevertheless, the mechanisms by which these signals are transduced are not yet known. In the current study, we conduct a two-stage GWAS on three myopia-related traits—axial length, spherical error and corneal curvature—within the Nagahama Prospective Genome Cohort for Comprehensive Human Bioscience (the Nagahama Study), which involves 9,804 healthy Japanese individuals. The analysis of an additional 2,674 Chinese individuals across two independent cohorts and 2,690 Caucasian individuals across five independent cohorts confirms the trans-ethnic genetic associations. In addition, we evaluate the associations with extreme myopia in Asian individuals. 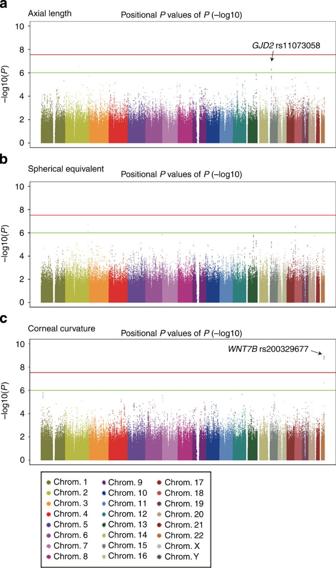Figure 1: Manhattan plots of the first stage GWAS for three myopia-related traits. Each plot shows −log10-transformedPvalues for all SNPs. The upper horizontal line represents the genome-wide significance threshold ofP<2.82 × 10−8, and the lower line represents the suggestive threshold ofP<1.00 × 10−6. Nine SNPs from five genes surpassed the suggestivePvalue, including previously reportedGJD2(P=4.72 × 10−7by linear regression using 2,991 individuals) for axial length and the novel genome-wide hitWNT7Bfor corneal curvature (Ptop=1.13 × 10−9by linear regression using 2,747). Two-stage GWAS within the Nagahama study The cohort demographics used in this study are shown in Supplementary Table 1 . After stringent quality control, a total of 1,773,334 single nucleotide polymorphisms (SNPs) were included in the analyses of the Nagahama cohort. Axial length, spherical equivalent and corneal curvature were used as the dependent variables for three genome-wide quantitative trait loci (QTL) analyses. We included age, sex and height as covariates, but did not include principal components in these analyses. However, inflation factors ( λ GC ) of 1.031 (axial length), 1.024 (spherical equivalent) and 1.016 (corneal curvature) indicated excellent control of population substructure. The QQ plots are shown in the Supplementary Fig. 1 . During the first stage, we identified five loci that showed a suggestive association with a P value <1.0 × 10 −6 by linear regression; one of these SNPs was WNT7B rs200329677, which exceeded genome-wide significance with a P value of 1.13 × 10 −9 in the association with corneal curvature ( Fig. 1 and Table 1 ). In the following replication stage, we further genotyped 3,460 Japanese individuals for three SNPs that showed suggestive association with a P value <1.0 × 10 −6 and had a minor allele frequency (MAF) of at least 5% in the discovery stage. 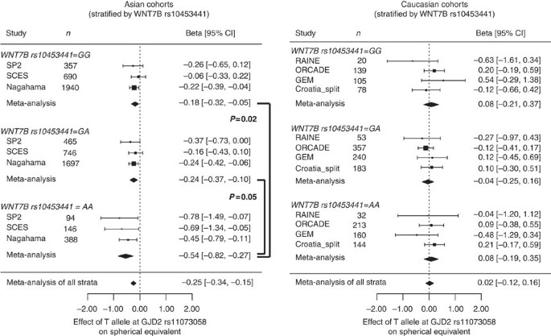Figure 2: Assessment of interactive effect betweenWNT7BandGJD2and association with the spherical equivalent. In Asian cohorts, the effects ofGJD2rs11073058 on the spherical equivalent were highest when the individual had the homozygous variant (AA genotype) atWNT7Brs10453441 (β=−0.54 D; 95% CI=−0.82 to −0.27 D), compared with individuals with the AG genotype (β=−0.24 D; 95% CI=−0.37 to −0.10 D;P=0.05 byz-test) or those with the GG genotype (β=−0.18 D; 95% CI=−0.32 to −0.05 D;P=0.02 byz-test). This trend was not observed in Caucasian cohorts. We investigated the associations of each of the three traits with each SNP and evaluated the results of the first and second stage in a meta-analysis ( Table 2 ). This analysis revealed associations with two traits for the two SNPs in GJD2 and WNT7B . First, we successfully replicated the previously reported association between GJD2 rs11073058 and axial length ( P combined =2.4 × 10 −8 ; inverse variance meta-analysis of discovery and replication results from Japanese cohort) as well as spherical equivalent ( P combined =2.7 × 10 −9 ). We did not observe any association between GJD2 rs11073058 and corneal curvature. Second, we confirmed the novel associations of WNT7B rs200329677 with corneal curvature ( P combined =2.5 × 10 −25 ) and axial length ( P combined =1.0 × 10 −8 ). This SNP did not show association with the spherical equivalent. Figure 1: Manhattan plots of the first stage GWAS for three myopia-related traits. Each plot shows −log 10 -transformed P values for all SNPs. The upper horizontal line represents the genome-wide significance threshold of P <2.82 × 10 −8 , and the lower line represents the suggestive threshold of P <1.00 × 10 −6 . Nine SNPs from five genes surpassed the suggestive P value, including previously reported GJD2 ( P =4.72 × 10 −7 by linear regression using 2,991 individuals) for axial length and the novel genome-wide hit WNT7B for corneal curvature ( P top =1.13 × 10 −9 by linear regression using 2,747). Full size image Table 1 Results of the discovery stage. Full size table Table 2 Results of the replication stage within the Nagahama Study ( n =3,460). Full size table Replication in other ethnicities and meta-analysis Of the current commercially available DNA microarrays, the WNT7B rs200329677 was included only on the Illumina HumanOmni 2.5 and 5 M chips. This SNP is not available in the 1000 Genomes Project or in the HapMap Project; thus, imputation to these reference genomes did not allow us to directly assess rs200329677 for association. Association with a trait was sought with rs10453441, which was in very high linkage disequilibrium with rs200329677 ( R 2 =0.967 in the Nagahama Study data set), and strong evidence was found for association to corneal curvature ( P discovery =2.16 × 10 −9 and P replication =4.6 × 10 −17 in the Nagahama data sets). We conducted replication of both SNPs in an additional 2,674 Chinese individuals across two independent collections, as well as across 2,835 Caucasian individuals across five collections ( Supplementary Methods ). 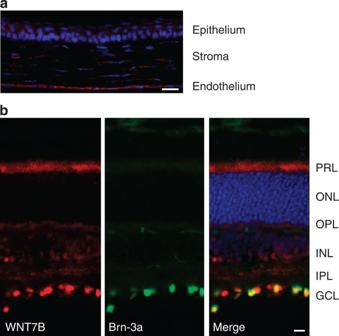Figure 3: Expression of WNT7B in retinal ganglion cells of C57BL/6 mice. (a) Mouse corneal sections were immunostained with antibodies against WNT7B (red). The upper part of the panel shows the corneal epithelium. (b) Mouse retinal sections were immunostained with antibodies against WNT7B (red) and Brn-3a (green). The nuclei are counterstained with 4′,6-diamidino-2-phenylindole (blue) in the merged image. The upper part of the panel shows the retinal pigment epithelium side, while the lower panel shows the vitreous side. WNT7B expression was observed in ganglion cells stained with Brn-3a. Scale bar, 10 μm. GCL, ganglion cell layer; INL, inner nuclear layer; IPL, inner plexiform layer; ONL, outer nuclear layer; OPL, outer plexiform layer; PRL, photoreceptor layer. The SNP rs10453441 showed significant evidence of replication ( Table 3 ) for axial length and corneal curvature both in Asian ( P AL =7.1 × 10 −6 , P CC =3.0 × 10 −14 ) and, to a lesser extent, in Caucasian ( P AL =2.0 × 10 −3 , P CC =4.1 × 10 −2 ) groups, with no heterogeneity across the two collections of Asian individuals ( I 2 AL =0, I 2 CC =0) and moderate-to-high heterogeneity across the five collections of Caucasian individuals ( I 2 AL =0.38, I 2 CC =0.89). Meta-analysis of the data from all the Asian collections showed genome-wide significant associations with both axial length ( P meta-Asian =1.20 × 10 −9 , β =0.129 mm) and corneal curvature ( P meta-Asian =9.00 × 10 −39 , β =0.053 mm), with no evidence of heterogeneity. Table 3 Replication of the association of WNT7B SNPs with three traits. Full size table Finally, meta-analysis of the Asian and Caucasian data also revealed strong associations between WNT7B rs10453441 and axial length ( P meta-ALL =3.9 × 10 −9 , β =0.121±0.017 mm), as well as corneal curvature ( P meta-ALL =2.7 × 10 −40 , β =0.051±0.004 mm). Only in the Genes in Myopia cohort [22] could we obtain Caucasian genotypes for both rs10453441 and rs200329677, so that we could assess the linkage disequilibrium (LD) between these two SNPs in Caucasians. They were in moderate LD ( R 2 =0.499, D ′=0.943). Possible interactive effect of WNT7B and GJD2 GJD2 is an established susceptibility gene for increased axial length and myopic refraction [11] , [23] . In the current study, these associations with GJD2 were replicated in our independent Japanese sample collections. To further our understanding of the role of GJD2 and WNT7B , we investigated the potential interactive effect of these two genes on myopia susceptibility by the directly genotyped cohorts: Nagahama replication samples, SCES, SP2, Raine, Croatia-split, ORCADES and Genes in Myopia. Figure 2 shows the effect of the GJD2 rs11073058 T allele on spherical equivalent, stratifying by the genotypes of WNT7B rs10453441. As described in Fig. 2 , in the Asian populations, the effects of GJD2 rs11073058 on spherical equivalent were the highest when individuals were homozygous (AA genotype) at WNT7B rs10453441 ( β =−0.54 D; 95% CI: −0.82 to −0.27 D) compared with that in the individuals with the AG genotype ( β =−0.24 D; 95% CI: −0.37 to −0.10 D) or in those with the GG genotype ( β =−0.18 D; 95% CI: −0.32 to −0.05 D). The genotypic model revealed marginal effect-measure modification ( P genotypic (analysis of variance) =0.07), with post hoc P values of 0.02 (AA versus GG), 0.05 (AA versus AG) and 0.60 (AG versus GG) based on z -test. On the other hand, the recessive model of effect-measure modification was statistically significant ( P recessive =0.024) as the effect of GJD2 rs11073058 T allele on spherical equivalent was −0.21 D (95% CI: −0.11 to −0.31 D) in individuals with non-AA genotype at WNT7B rs10453441. Figure 2: Assessment of interactive effect between WNT7B and GJD2 and association with the spherical equivalent. In Asian cohorts, the effects of GJD2 rs11073058 on the spherical equivalent were highest when the individual had the homozygous variant (AA genotype) at WNT7B rs10453441 ( β =−0.54 D; 95% CI=−0.82 to −0.27 D), compared with individuals with the AG genotype ( β =−0.24 D; 95% CI=−0.37 to −0.10 D; P =0.05 by z -test) or those with the GG genotype ( β =−0.18 D; 95% CI=−0.32 to −0.05 D; P =0.02 by z -test). This trend was not observed in Caucasian cohorts. Full size image Clinical relevance of WNT7B to extreme myopia To evaluate the possible association between WNT7B and extreme myopia, we performed a case–control study. We found significant association between WNT7B rs10453441 and extreme myopia (patients with average axial length of ≥28 mm) in the Japanese cohort (odds ratio=1.14 (95% CI=1.02–1.27), P meta-Japanese =0.018). Although the association in Chinese cohorts was not statistically significant ( P meta-Chinese =0.30), the effect size and its direction were similar to those in Japanese cohort (odds ratio=1.10 (95% CI=0.92–1.30)). The lack of association might be due to the limited sample size of extreme myopia individuals (1,064 Japanese and 414 Chinese) as these results were consistent ( I 2 =0%, P heterogeneity =0.84). Indeed, overall meta-analysis revealed more significant association (odds ratio=1.13 (95% CI=1.03–1.24), P meta-all =0.011). 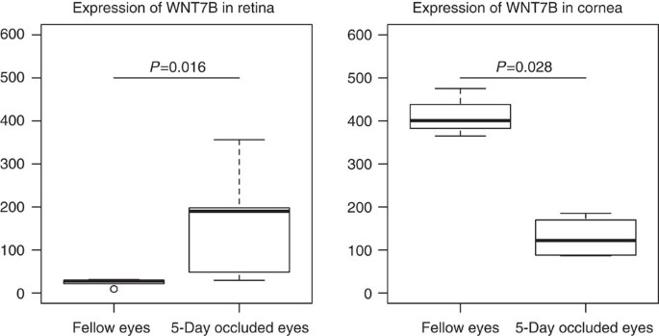Figure 4: Differential expression of WNT7B between treated eyes and fellow eyes in experimental myopia mice (n=5 in each arm). The vertical axis indicates WNT7B expression normalized to β-actin expression. WNT7B expression in the retina was significantly upregulated in the experimental myopia eyes (P=0.016 by Wilcoxon test), but was significantly downregulated in the cornea (P=0.028 by Wilcoxon test). These results are summarized in Table 4 and Supplementary Fig. 2 . Table 4 Association of WNT7B rs10453441 with extreme myopia. Full size table The expression of WNT7B in experimental myopia mice Our immunohistochemical study of the mouse cornea showed that WNT7B was predominantly expressed in the endothelial cell layer ( Fig. 3a ). In contrast to corneal studies, the role of WNT signaling in the posterior pole has been examined in various parts of the tissue, such as the neural retina, retinal vasculature and retinal pigment epithelium [24] , [25] , [26] , [27] , [28] . To evaluate the expression pattern of WNT7B in the posterior pole of eyes, we examined the localization of WNT7B in the mouse eye. In the retina of a 21-day-old male mouse, WNT7B expression was observed predominantly in ganglion cells ( Fig. 3b ). Ganglion cells were also stained with the ganglion cell marker Brn-3a. Not all ganglion cells expressed Brn3a, and hence we could not confirm expression of WNT7B in all ganglion cells, but we could confirm that all ganglion cells expressing Brn-3a also co-expressed WNT7B. Figure 3: Expression of WNT7B in retinal ganglion cells of C57BL/6 mice. ( a ) Mouse corneal sections were immunostained with antibodies against WNT7B (red). The upper part of the panel shows the corneal epithelium. ( b ) Mouse retinal sections were immunostained with antibodies against WNT7B (red) and Brn-3a (green). The nuclei are counterstained with 4′,6-diamidino-2-phenylindole (blue) in the merged image. The upper part of the panel shows the retinal pigment epithelium side, while the lower panel shows the vitreous side. WNT7B expression was observed in ganglion cells stained with Brn-3a. Scale bar, 10 μm. GCL, ganglion cell layer; INL, inner nuclear layer; IPL, inner plexiform layer; ONL, outer nuclear layer; OPL, outer plexiform layer; PRL, photoreceptor layer. Full size image To explore the roles of WNT7B in myopia development, we evaluated the expression of the WNT7B gene in the cornea and the neural retina of myopia-induced mice ( Fig. 4 ). WNT7B mRNA levels were significantly higher in the retinas of myopic eyes than those of corresponding control eyes ( P =0.016). In contrast, WNT7B mRNA levels were significantly reduced in the corneas of myopic eyes ( P =0.029). Figure 4: Differential expression of WNT7B between treated eyes and fellow eyes in experimental myopia mice ( n =5 in each arm). The vertical axis indicates WNT7B expression normalized to β-actin expression. WNT7B expression in the retina was significantly upregulated in the experimental myopia eyes ( P =0.016 by Wilcoxon test), but was significantly downregulated in the cornea ( P =0.028 by Wilcoxon test). Full size image We performed a GWAS in a large Japanese cohort and found that WNT7B was significantly associated with axial length and corneal curvature. The associations with axial length and corneal curvature were successfully replicated in both Chinese and Caucasian cohorts. In addition, the WNT7B genotype strengthened the effects of GJD2 , a widely replicated myopia susceptibility gene [11] , [23] . Furthermore, the WNT7B polymorphism rs10453441 was also significantly associated with extreme myopia. Our findings that WNT7B expression was downregulated in the cornea and upregulated in retinal ganglion cells in experimental myopia suggested that WNT7B plays a key role in controlling myopia development through compensatory mechanisms. Although many candidate gene studies [29] , [30] , [31] , [32] , [33] and GWASs [10] , [11] , [12] , [34] , [35] , [36] , [37] , [38] , [39] have been conducted to investigate myopia-associated traits, little is known about the pivotal pathways involved in the development of myopia. The largest genome-wide meta-analysis conducted by CREAM [11] on refractive error and a recent large GWAS conducted by 23andMe [39] on age of myopia onset reported a total of 42 loci associated with myopia. Many of them were associated with signaling cascades in the neural retina, retinal pigment epithelium, choroid and sclera. However, not all the susceptibility genes were detected by previous GWASs because it is difficult to detect SNPs with low minor-allele frequencies or small effect sizes and because SNPs that were not included in the commercially available assay could not be evaluated. Even though a genomic imputation technique was used, the imputation quality was not necessarily high as it is dependent on whether imputed SNPs are in high LD with directly genotyped SNPs. To overcome this problem, we applied the dense 2.5 M chip for 53.7% of the samples and a 610 K chip for 49.3% of the samples, which were imputed to the intra-cohort reference panel (296 samples from the Nagahama Study cohort genotyped using all platforms). This strategy provided a dense, high-quality data set and enabled us to find a novel susceptibility gene for corneal curvature and axial length. The novel susceptibility gene, WNT7B , had stronger effects on axial length ( β =0.13) than the established susceptibility gene, GJD2 ( β =0.09 in the current study and β =0.06–0.07 in a previous report [12] ). Although the genotypes of the SNPs within WNT7B were not directly associated with refractive error in the Nagahama Study, which only included a small number of subjects with extreme myopia (49 individuals in first and second stage), SNPs within WNT7B displayed significant associations with extreme myopia in our case–control studies. These data suggest that the effects of WNT7B might become apparent when the compensatory mechanisms of eye components to control refractive error are disrupted, resulting in extreme myopia. Therefore, we investigated the interactive effect of WNT7B on GJD2 for refractive error. The effects of the T-risk allele of rs11073058 in GJD2 on myopia were the largest when the genotype of WNT7B rs10453441 was AA. As the reported effect size of GJD2 on refraction ranged from −0.10 D to −0.12 D (refs 12 , 40 ), the acceleration of myopia by WNT7B up to −0.54 D per copy of the T allele at GJD2 rs11073058 in Asians is of note, which is statistically significant in the recessive model. Interestingly, this interactive effect was not apparent in Caucasian samples. This might be due to the limited sample size of the Caucasian cohorts, allelic differences between Asians and Caucasians, or it might, in part, explain the higher prevalence of myopia in Asians. In a mouse model, WNT7B was downregulated in the cornea and upregulated in the retina of experimental myopic eyes. Considering that the effect of WNT7B rs10453441 on myopia through axial length is in the opposite direction to that through corneal curvature, WNT7B may be under strict control to correlate the anterior and posterior segments in the emmetropization of the eye. To date, accumulating evidence suggests that retinal image defocus is the trigger for myopia, and the role of amacrine cells in delivering an image defocus signal has been intensively investigated in the context of myopia development [20] , [21] , [41] . Nevertheless, the precise mechanisms mediating the transduction of this defocus signal leading to myopia are still unclear. GJD2 is reportedly localized at the synapses between alpha-ganglion cells, AII amacrine cells, cone bipolar cells and photoreceptor cells [42] , [43] , [44] , [45] , [46] , [47] , [48] , [49] , [50] , [51] . Of all the interactions between these cells, the coupling between the amacrine cells and ganglion cells has been reported to be dramatically reduced in GJD2 knockout mice [52] . Together with our findings indicating that WNT7B was localized to retinal ganglion cells and that its expression was significantly upregulated in experimental myopic eyes, these data support the hypothesis that WNT7B and GJD2 co-operatively regulate the normal growth of the eye through interactions between the alpha-ganglion cells and AII amacrine cells. Interestingly, alpha-ganglion cells are predominantly observed in the peripheral retina and have large dendritic regions to receive inputs from amacrine cells [47] , [53] , [54] , [55] , [56] , [57] . The hypothesis that alpha-ganglion cells and AII amacrine cells are implicated in emmetropization is consistent with the peripheral defocus theory, a theory of myopia development that has been supported by clinical evidence [58] , [59] , [60] , [61] . Although the current study revealed for the first time the possible involvement of WNT7B in myopia development, the involvement of Wnt signaling itself in this process has been suggested previously. For example, we showed that polymorphisms in PAX6 and δ-catenin ( CTNND2 ) are associated with high-grade myopia [29] , [32] , [33] , [35] . PAX6 can directly control both CTNND2 and WNT7B expression [62] , [63] , and both molecular pathways can result in increased β-catenin nuclear translocation to activate Wnt signaling [64] , [65] . Independently, the CREAM consortium found that polymorphisms in RSPO1 and ZNRF3 , which regulate Wnt signaling by controlling the turnover of Wnt receptors, were significantly associated with axial length [12] , [66] . The present study suggests that WNT7B can be involved in the development of myopia. Further studies are needed to investigate interactions between genes in the same or different cascades of Wnt-signaling pathways. Better understanding of the pathophysiology underlying myopia will guide interventions for prevention and treatment. In summary, we have demonstrated significant association of WNT7B with corneal curvature and axial length in three different ethnic groups and found that WNT7B could facilitate the development of myopia through cooperation with GJD2 . Furthermore, the WNT7B polymorphism rs10453441 was significantly associated with extreme myopia in patients with Asian ancestry. In the retina, WNT7B was localized to ganglion cells, and its expression was significantly increased in mice with experimental myopia, whereas in the cornea its expression was localized to the endothelium and its expression downregulated in experimental myopia. We, therefore, propose that Wnt-signaling pathways that are vital for coordinating vision and disruption in these pathways leads to myopia. Patient enrollment There were 9,804 Japanese participants in the Nagahama Prospective Genome Cohort for Comprehensive Human Bioscience (the Nagahama Study). The Nagahama Study cohort was recruited from 2008 to 2010 from the general population living in Nagahama City, Shiga Prefecture, Japan [67] , [68] . All ophthalmological measurements and blood sampling were performed at the time of enrollment. Genomic DNA was extracted from peripheral blood samples by the phenol–chloroform method. All study procedures were approved by the Ethics Committee of Kyoto University Graduate School of Medicine. For the replication stage, we also included seven other cohorts that consisted of five Caucasian cohorts and two Singaporean Chinese cohorts. Detailed information and sample collections for these cohorts can be found in the Supplementary Methods . All patients were enrolled in the study after giving informed consent, ethical approval was granted by the SingHealth Centralized Institutional Review Board (cohorts SP2 and SCES), the Ethics Committee of the Medical School, University of Split and the NHS Lothian South East Scotland Research Ethics Committee (CROATIA-Split and CROATIA-Korcula) and the NHS Orkney Research Ethics Committee and the North of Scotland Research Ethics Committee (ORCADES). The Human Research and Ethics Committee of the Royal Victorian Eye and Ear Hospital, Melbourne (GEM) and the King Edward Memorial Hospital and Princess Margaret Hospital for Children ethics boards (RAINE). Genomic DNA was extracted from peripheral blood samples according to standard laboratory procedures. Individuals who had undergone ocular surgery (with the exception of cataract surgery) and who had undergone ocular laser treatment were excluded from the analysis of all three traits. In addition, individuals who had undergone cataract surgery were excluded from analyses of the spherical equivalent and corneal curvature. Evaluation of ophthalmological measurements All the participants in the Nagahama Study had their axial length (millimeter (mm); IOL Master, Carl Zeiss Meditec, Dublin, CA, USA), spherical equivalent (diopter (D); ARK-530A, Nidek, Aichi, Japan) and corneal curvature (mm; ARK-530A, Nidek) measured for both eyes. Colour fundus photographs were also obtained from all the participants (CR-DG10, Canon, Tokyo, Japan). History of cataract surgery, ocular surgery other than cataract surgery and ocular laser treatment, including photocoagulation, was obtained using a questionnaire. For the replication cohorts, detailed information is given in the Supplementary Methods . Genome-wide SNP genotyping Genome-wide SNP genotyping was performed on samples from 3,710 participants who joined the Nagahama cohort from 2008 to 2009. A series of BeadChip DNA arrays, namely HumanHap610 Quad (1,828 samples), HumanOmni2.5-4 (1,616 samples), HumanOmni2.5-8 (378 samples), HumanOmni2.5s (192 samples) and HumanExome (192 samples; Illumina, San Diego, CA, USA) were used for the analysis. Some of the samples were repeatedly genotyped using different arrays, and 296 samples that had been genotyped using HumanHap610 Quad, HumanOmni2.5-8, HumanOmni2.5s and HumanExome were used as a reference panel in the genotype imputation. SNPs with a call rate <99%, MAF <1% and significant deviation from Hardy–Weinberg Equilibrium ( P value for deviation <1.0 × 10 −7 ) were excluded from further statistical analysis. Samples with a call rate <95% ( n =162) were excluded from the analysis. Among the remaining 3,548 subjects, 295 estimated to have a first- or second-degree kinship within this population (pi-hat >0.35, PLINK ver. 1.07 ( http://pngu.mgh.harvard.edu/~purcell/plink/ )) and seven ancestry outliers identified by principal component analysis with the HapMap Phase 2 release 28 JPT data set as a reference (EIGENSTRAT ver. 2.0 ( http://www.hsph.harvard.edu/alkes-price/software/ )) were also excluded from the analysis. Genotype imputation was performed using MACH ver. 1.0.16 software ( http://www.sph.umich.edu/csg/abecasis/MACH/tour/imputation.html ) and 1,792,015 SNPs from the 296-sample reference panel. Imputed SNPs for which the MAF was <0.01% or R 2 <0.5 were excluded from the following association analysis. Finally, 1,773,334 SNPs from 3,248 individuals were fixed. Replication genotyping We conducted a two-stage replication study. The first stage was the replication within the Nagahama Study participants and the second stage was the trans-ethnic replication. For the first stage, we genotyped the subset of remaining samples from the Nagahama Study ( n =3,460) whose phenotypes were all available using TaqMan allelic discrimination probes (Applied Biosystems). For the second stage, genotypes of rs200329677 and/or rs10453441 were determined by one of the following methods: using the HumanOmni1M chip (Illumina), using TaqMan allelic discrimination probes (Applied Biosystems) or imputation from the existing data. The particular method used is described in Supplementary Table 2 . We first used direct genotyping data. However, if only imputed data were available, we included them only when the imputation quality ( R 2 ) was >0.5. Statistical analysis Genome-wide QTL analysis was conducted for the three myopia-related traits: axial length, spherical equivalent and corneal curvature. We used the mean values of both eyes for each trait. If one eye was not applicable, measurement of the other eye was used in the analysis. For every post-QC SNP, we evaluated the association between the genotypes and the trait using a multivariable linear regression, assuming an additive model. This regression framework allowed us to adjust for covariates such as age, sex and height. Experimental-wide significance was set at 2.82 × 10 −8 , corresponding to P =0.05 divided by the 1,773,334 SNPs included in the QTL analysis. We also carried SNPs with P values <1.00 × 10 −6 forward to the replication stage if their MAFs were at least 5%. Meta-analysis was conducted using inverse variance weights for 8,981 Asians, 2,835 Caucasians and all subjects. This process was performed using the METAL software ( http://www.sph.umich.edu/csg/abecasis/Metal/ ). Estimates of effect size with standard error were compared using the z -test. Manhattan plots and forest plots (package ‘metafor’) were generated using R version 2.15 ( http://www.r-project.org ). Association with extreme myopia To investigate the association between WNT7B rs10453441 and extreme myopia, we performed two association tests. In these analyses, we defined extremely myopic patients as patients whose average axial lengths in both eyes were >28.00 mm, according to a previous report [9] . Samples whose average axial lengths ranged from 22.00 to 24.00 mm were used as control samples. We used two case–control data sets of the Japanese population. The first one was the Kyoto/Nagahama data set consisting of 938 highly myopic cases recruited from the Kyoto High Myopia cohort [9] , [29] , [30] and 1,902 controls extracted from the Nagahama Study samples genotyped by the TaqMan method. The Kyoto High Myopia samples were also genotyped using the TaqMan method. The second cohort consisted of Yokohama samples, recruited from Yokohama City University, which contained 109 extreme myopia patients and 395 controls. They were both genotyped using Illumina OmniExpress at Yokohama City University. The demographics of the Kyoto High Myopia cohort and the Yokohama samples are shown in Supplementary Table 3 . For further replication, three Chinese cohorts, that is, SCES, Hong Kong and Sichuan, were used for the same analysis. Chinese samples were also genotyped using the TaqMan method. The analyses were performed using logistic regression. Meta-analyses were conducted using inverse-variance weights for two Japanese cohorts, three Chinese cohorts and all five cohorts. Experimental myopia mouse model To induce form-deprivation myopia in mice [16] , [69] , [70] , we occluded the right eyes of male C57BL/6 mice (Japan SLC Inc., Shizuoka, Japan) with diffuser goggles from postnatal day 21. The mice were housed individually in standard mouse cages for 5 days at 25 °C on a 12 h:12 h light:dark cycle, with standard rodent chow pellets and water freely available. The animal study was approved by the Kyoto University Animal Experimentation Committee. All the procedures performed in this study complied with the Association of Research in Vision and Ophthalmology Statement for the Use of Animals in Ophthalmology and Vision Research. Immunohistochemical staining After a mouse was killed, eyes were enucleated and fixed with 4% paraformaldehyde in 0.1 M PB for 20 min. The expression of WNT7B in the retina was examined in vertical sections. For this, the eyes were cryoprotected in a sucrose gradient (10 and 30% w/v sucrose in 0.1 M PB), and 14-μm cryostat sections were cut. The sections were blocked for 1 h in a solution containing 10% normal goat serum (Millipore), 0.3% Triton X-100 (Bio-Rad, Hercules, CA, USA) and 0.1 M PB. The primary antibodies were diluted in the blocking solution and incubated overnight at 4 °C, followed by incubation for 1 h in the secondary antibody solution. The primary antibodies used were 1:200 dilution of rabbit anti-Wnt7b (NOVUS, NBP1-59564) and 1:100 dilution of mouse anti-Brn-3a (CHEMICON, MAB1585). For secondary antibodies, 1:1,000 dilutions of Alexa Fluor 594 goat anti-rabbit IgG (H+L) and Alexa Fluor 488 goat anti-mouse IgG (H+L) antibodies (catalogue numbers A-11012 and A-11001, respectively, Invitrogen, Eugene, OR, USA) were used. All the steps were carried out at 4 °C. All the images were obtained using a KEYENCE BZ-9000 microscope. Quantitative real-time polymerase chain reaction To evaluate changes in the expression level of WNT7B at the early stage of myopia, we used experimental mice treated for 5 days. Gene expression in the corneas and retinas of treated and untreated eyes were compared using a Wilcoxon test. Total RNA was isolated from mouse corneas or neural retinas using QIAzol Reagent (Qiagen, Tokyo, Japan) for the experimental eyes ( n =5) and untreated eyes ( n =5). RNA was purified using the RNeasy Micro kit (Qiagen). Purified RNA was reverse transcribed into cDNA by using a ReverTra Ace quantitative real-time polymerase chain reaction (qPCR) RT Kit (Toyobo, Hiroshima, Japan). We performed qPCR using ThunderBird SYBR qPCR mix (Toyobo) to validate the gene expression. The sequences of the qPCR primers are shown in Supplementary Table 4 . The reactions were run using an ABI Prism 7300 Sequence Detection System (Applied Biosystems, Foster City, CA, USA) for 40 cycles under the following conditions: 95 °C for 15 s and 60 °C for 60 s. To normalize for input load of cDNA between samples, β-actin was used as an endogenous internal control. Threshold cycle (CT) was determined automatically, and relative change in mRNA expression was calculated using ΔΔCT values. All cDNA samples were tested in triplicate and the average values were used in statistical analysis. How to cite this article: Miyake, M. et al. Identification of myopia-associated WNT7B polymorphisms provides insights into the mechanism underlying the development of myopia. Nat. Commun. 6:6689 doi: 10.1038/ncomms7689 (2015).